CMOS-based carbon nanotube pass-transistor logic integrated circuits Field-effect transistors based on carbon nanotubes have been shown to be faster and less energy consuming than their silicon counterparts. However, ensuring these advantages are maintained for integrated circuits is a challenge. Here we demonstrate that a significant reduction in the use of field-effect transistors can be achieved by constructing carbon nanotube-based integrated circuits based on a pass-transistor logic configuration, rather than a complementary metal-oxide semiconductor configuration. Logic gates are constructed on individual carbon nanotubes via a doping-free approach and with a single power supply at voltages as low as 0.4 V. The pass-transistor logic configurarion provides a significant simplification of the carbon nanotube-based circuit design, a higher potential circuit speed and a significant reduction in power consumption. In particular, a full adder, which requires a total of 28 field-effect transistors to construct in the usual complementary metal-oxide semiconductor circuit, uses only three pairs of n- and p-field-effect transistors in the pass-transistor logic configuration. Semiconducting carbon nanotubes (CNTs) are considered to be promising channel materials for the next-generation nanoelectronic devices, in particular, for high-performance field-effect transistors (FETs) [1] , [2] , [3] . After approximately 15 years of extensive investigation, significant progress has been made in the fabrication of CNT-based nanoelectronic devices [1] , [2] , [3] , and the physics of the CNT FET has been firmly established [4] , [5] , [6] , [7] . Both p-type [8] , [9] , [10] , [11] and n-type [12] , [13] , [14] , [15] , [16] CNT FETs have been fabricated, displaying outstanding performance approaching the ballistic limit [11] , [13] , [14] . However, progress in developing CNT FET-based integrated circuits (ICs) has been slow. Although several basic logic gates, including NOT, NAND, NOR, AND, OR [17] , [18] , [19] , [20] , and the more complex five-stage ring oscillator have been fabricated [21] , CNT-based logical circuits that are more complex than an XOR gate have not been realised [22] , [23] , [24] , [25] . In particular, a CNT-based full adder, which is a basic function block in the arithmetic logic unit (ALU) of the modern digital computer [26] , has not been constructed. In addition to the well-known challenges related to construction materials, such as controlling position and chirality during CNT growth, CNT-based nanoelectronic circuits have scarcely been considered at the architectural level, and many important questions remain unanswered. Of particular interest is the problem of determining the most suitable circuit design configuration for CNT-based ICs [27] , [28] , [29] . An ideal design configuration for CNT-based ICs should fulfill at least the following two requirements. The first and most fundamental requirement is that circuit blocks designed with such a circuit configuration must possess sufficient signal gain and driving ability to guarantee signal fidelity and propagation in the circuit. The second requirement is that the design configuration should take the full advantage of the superb properties of CNT FETs and use as few transistors as possible while operating at higher speed and/or with lower power dissipation than conventional complementary metal-oxide semiconductor (CMOS) configurations. In this article, we focus on exploring a suitable circuit design configuration for CNT-based ICs, and constructing basic gates and more complex circuits for an ALU. At the physical level, high-performance CNT-based FETs are fabricated via a doping-free approach [12] . At the architectural level, CNT-based ICs are designed following the configuration of a pass-transistor logic (PTL), which significantly reduces the number of transistors required [27] , [28] , [29] . However, conventional Si-based PTL circuits encountered two major drawbacks; namely, threshold voltage drop and loss of gain, which have so far prevented PTL circuits from being widely used in ICs [29] . Here we show that both drawbacks can be eliminated in CNT-based PTL circuits via threshold voltage engineering and combining PTL circuits with CMOS inverters. Basic logic gates such as OR and AND, as well as the more complex full adder, multiplexer (MUX) and demultiplexer (DEMUX) circuits are successfully fabricated on individual CNTs for the first time. In addition, benefitting from the improved immunity of PTL circuits to threshold voltage fluctuations, CNT-based circuits with gate lengths of 1 μm can be powered by a single power supply operating at a voltage as low as 1 V, or even 0.4 V in some cases. Device fabrication and characterisation All the CNT-based FETs used in this work are fabricated on individual single-walled CNTs (SWCNTs) via a doping-free process [12] . A previously developed self-aligned top-gate structure [13] is used for the fabrication of both n-type and p-type FETs ( Fig. 1a ), where the polarity is determined by the contact metal, that is, Sc for n-type [12] and Pd for p-type CNT FETs [9] . As the conduction and valence bands of a semiconducting CNT are symmetric near the Fermi level, and the carrier injection efficiency is at the same level for both n- and p-contacts [20] , n-type and p-type CNT FETs show nearly symmetric electronic characteristics ( Fig. 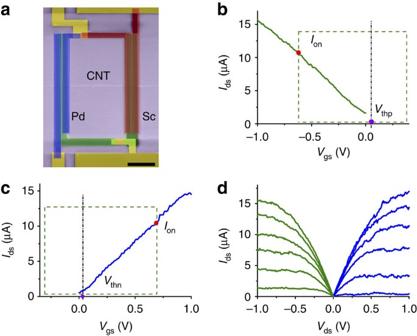Figure 1: Geometry and characteristics of the CNT-based FETs. (a) A scanning electron microscopic image showing a pair of p- and n-FETs on a single CNT, scale bar is 10 μm. Shown in (b) and (c) are the transfer characteristics of the p-FET and n-FET, based on the same CNT with a diameter of approximately 1.8 nm and a channel length of approximately 1 μm. For the p-FET, the source is biased at 1.0 V and drain is at 0 V, whereas for the n-FET, the source is biased at 0 V and the drain is at 1.0 V. The olive box defines the 1 V gate voltage window used to obtainIon, whereVthis determined using the standard peak transconductance method. The extractedVth(violet point) andIon(red point) are (b) 0.05 V and 10.6 μA for the p-FET, and (c) 0.03 V and 10.4 μA for the n-FET. (d) The output characteristics of the p-type (green lines) and n-type (blue lines) CNT FETs with |Vgs| varying from 0 to 1 V in steps of 0.2 V, from bottom to top. 1b–d ) and simultaneously high performance, including peak transconductances greater than 15 μS and saturation currents up to 15 μA at a bias of 1.0 V. The output characteristics of these devices are presented in Figure 1d , which illustrates the almost symmetric I ds − V ds curve for a pair of p- and n-FETs under various gate voltages ranging from 0 to 1.0 V in steps of 0.2 V. The intrinsic speed of the FETs is generally described by the performance metric of gate delay, defined as τ =CV/I, in which C is the total gate capacitance, V = V ds is the applied voltage, and I = I on is the ON-state current [30] . Here, the semiconducting CNT channel has a diameter (d) of 1.8 nm, and the gate dielectric HfO 2 thin film has a thickness ( t ) of 12 nm and an ɛ r of 18; we thus obtain C =1.71 pF cm −1 . The threshold voltage V th is extracted from Figure 1b and c (using the peak transconductance method [30] ), and found to be 0.05 V for the p-FET and 0.03 V for n-FET. By constructing a V DD (1.0 V) window, as illustrated in Figure 1b and c at V th , we thus obtain I on =10.6 μA for the p-FET and 10.4 μA for the n-FET at V ds =1.0 V. The intrinsic gate delay time of both the p-FET and n-FET with L g =1 μm is approximately 16 ps, which is comparable to that of the silicon NMOS devices with L g =0.5 μm. It should be noted that to obtain a suitable threshold voltage, Pd metal was used as the top gate, which effectively adjusted the threshold voltage of both the n-type and p-type FETs to centre it near 0 V for | V ds |=1 V ( Fig. 1b and c ). The high-performance and symmetric n-type and p-type CNT FETs with suitable threshold voltages thus provide the ideal building blocks for constructing CNT-based ICs, and in this work, all the circuits are designed and constructed to work with a single power supply providing V DD =1 V or 0.4 V. Figure 1: Geometry and characteristics of the CNT-based FETs. ( a ) A scanning electron microscopic image showing a pair of p- and n-FETs on a single CNT, scale bar is 10 μm. Shown in ( b ) and ( c ) are the transfer characteristics of the p-FET and n-FET, based on the same CNT with a diameter of approximately 1.8 nm and a channel length of approximately 1 μm. For the p-FET, the source is biased at 1.0 V and drain is at 0 V, whereas for the n-FET, the source is biased at 0 V and the drain is at 1.0 V. The olive box defines the 1 V gate voltage window used to obtain I on , where V th is determined using the standard peak transconductance method. The extracted V th (violet point) and I on (red point) are ( b ) 0.05 V and 10.6 μA for the p-FET, and ( c ) 0.03 V and 10.4 μA for the n-FET. ( d ) The output characteristics of the p-type (green lines) and n-type (blue lines) CNT FETs with | V gs | varying from 0 to 1 V in steps of 0.2 V, from bottom to top. Full size image CNT-based PTL circuits A popular and widely used alternative to the conventional CMOS logic configuration is the PTL configuration, which can significantly reduce the number of transistors required to implement a logic circuit and has the additional advantage of lower capacitance [27] , [28] , [29] . 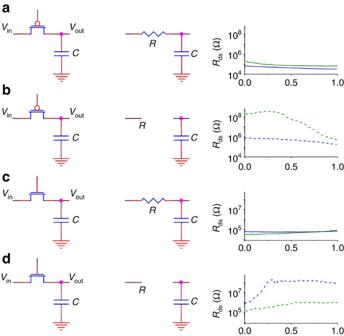Figure 2: The operating principles of CNT-based PTL circuits. Shown in (a) and (b) are schematic diagrams (left) depicting the operating principles and experimentally measured output resistances (right) of a p-type pass-transistor (a) in the ON state, that is, biasing the gate at 0 V and (b) in the OFF state, that is, biasing the gate at 1 V, respectively. In the right panels, the blue curves denote passing a logic '1', and the olive curves denote passing a logic '0'. The dotted lines represent the case of the OFF state, whereas the solid lines represent the case of the ON state. Shown in (c) and (d) are schematic diagrams (left) depicting the operating principles and experimentally measured output resistances (right) of an n-type pass-transistor (c) in the ON state, that is, biasing the gate at 1 V and (d) in the OFF state, that is, biasing the gate at 0 V, respectively. In the right panels, the green curves denote passing a logic '0', and the blue curves denote passing a logic '1'. The solid lines represent the case of the ON state, whereas the dotted lines represent the case of the OFF state. To measure the passing of a logic '1',Vinis set to 1.0 V. Conversely, to measure the passing of a logic '0',Vinis set to 0 V. Figure 2 illustrates the operating principles and experimental results for the PTL circuits using both p-type and n-type CNT FETs. For a p-type pass transistor ( Fig. 2a and b ), when a low voltage (a logic '0', or 0 V here) is applied to the gate ( Fig. 2a ), the resistance between the source (input) and drain (output) of the device, R ds , is on the order of 100 kΩ or less. The device is thus in its 'low-resistance' or 'ON' state, and may pass the input signal V in from the source to the drain. When a high bias (a logic '1', that is, 1.0 V here) is applied to the gate ( Fig. 2b ), R ds is greater than 500 kΩ. The p-type device is thus in its 'high-resistance' or 'OFF' state and may not pass the input signal V in to the output faithfully. The operation of an n-type pass transistor is similar to that of a p-type pass transistor, but in a complementary way. The n-type pass transistor can pass an input signal when a logic '1' is biased on the gate ( Fig. 2c ), and it is turned off when a logic '0' is biased on the gate ( Fig. 2d ). It should be noted that pass transistors are used here as switches to pass logic levels between the nodes of a circuit, rather than as switches connected directly to the power supply. Figure 2: The operating principles of CNT-based PTL circuits. Shown in ( a ) and ( b ) are schematic diagrams (left) depicting the operating principles and experimentally measured output resistances (right) of a p-type pass-transistor ( a ) in the ON state, that is, biasing the gate at 0 V and ( b ) in the OFF state, that is, biasing the gate at 1 V, respectively. In the right panels, the blue curves denote passing a logic '1', and the olive curves denote passing a logic '0'. The dotted lines represent the case of the OFF state, whereas the solid lines represent the case of the ON state. Shown in ( c ) and ( d ) are schematic diagrams (left) depicting the operating principles and experimentally measured output resistances (right) of an n-type pass-transistor ( c ) in the ON state, that is, biasing the gate at 1 V and ( d ) in the OFF state, that is, biasing the gate at 0 V, respectively. In the right panels, the green curves denote passing a logic '0', and the blue curves denote passing a logic '1'. The solid lines represent the case of the ON state, whereas the dotted lines represent the case of the OFF state. To measure the passing of a logic '1', V in is set to 1.0 V. Conversely, to measure the passing of a logic '0', V in is set to 0 V. Full size image The main advantage of using PTL is that one pass transistor (either a p-type or an n-type) is sufficient to perform a logical operation, which greatly reduces the number of transistors used compared with a circuit using a conventional CMOS configuration to achieve the same function [29] . One major drawback in the Si-based PTL is that although an n-type pass transistor may produce a 'strong zero' or ground, it produces only a 'weak one' by lowering the output below V DD − V thn , where V thn is the threshold voltage of the n-FET. In contrast, a p-type pass transistor produces a 'strong one', but a 'weak zero' by raising the output above | V thp | when the input is zero, where V thp is the threshold voltage of the p-FET. This drawback results from different threshold voltages for n-type and p-type FETs, and the change in the output is usually referred to as threshold voltage drop [27] , [28] , [29] . One possible solution to this problem is to adjust the threshold voltages of both the n-type and p-type FETs, such that V thn ≈ V thp ≈0 at the processing level via doping. However, this is usually not desirable in conventional Si CMOS technology [29] . By contrast, the threshold voltage is readily adjustable in doping-free CNT CMOS technology [13] , [21] . Supplementary Fig. S1 demonstrates that it is possible to move the threshold voltage of both n-type and p-type FETs to centre them at approximately 0 V by selecting a suitable gate metal, which significantly reduces the conventional threshold voltage in CNT FET-based PTL circuits. However, finite threshold voltage drops for both the n-type and p-type CNT FETs as pass transistors still exist, as implied in Figure 2 . For a p-type FET ( Fig. 2a ), the output resistance for passing a logic '0' in its 'ON' state (the solid green line) is obviously larger than that for passing a logic '1' (the solid blue line). Therefore, there still exists a small threshold voltage drop for the p-type CNT FET when a logic '0' is passed, and the voltage drop is significantly lower when passing a logic '1'. Similarly, an n-type FET passes a logic '0' well, while passing a logic '1' with an obviously larger R ds or threshold drop at low bias ( Fig. 2c ). However, benefitting from the small threshold voltage near zero, the threshold voltage drops for both n-type and p-type CNT pass transistors are much smaller than their conventional silicon counterparts, which show threshold voltages that are typically ten times larger [31] . On the basis of these high-performance CNT pass transistors, many types of high-performance logic ICs can thus be designed and built with a PTL configuration. Basic logic gates We first consider the OR gate. 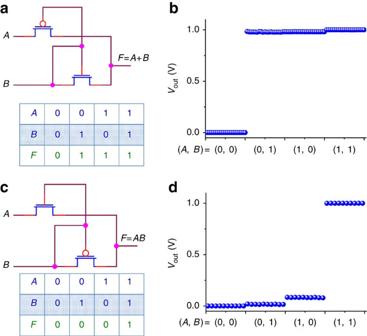Figure 3: CMOS-based pass-transistor OR and AND gates. (a) Circuit design (top) and truth table (bottom) for an OR gate. (b) Output voltage levels for all four input states of the OR gate. (c) Circuit design (top) and truth table (bottom) for an AND gate. (d) Output voltage levels for all four input states of the AND gate. Figure 3a is a circuit diagram designed with a PTL configuration together with a truth table for the OR gate. The outputs for all four ( A , B ) input combinations are shown in Fig. 3b , illustrating an excellent OR logic function. Among the four outputs, those corresponding to the input combinations ( A , B )=(0, 0) and (1, 1) are almost perfect, whereas the outputs for the input combinations ( A , B )=(0, 1) and (1, 0) are 0.96 V and 0.97 V, respectively, for a power supply of V DD =1 V, and are thus slightly degraded. The output voltage drop for each input combination depends mainly on the threshold voltages of the involved CNT FETs and can be estimated from the output characteristics of the device. Figure 3: CMOS-based pass-transistor OR and AND gates. ( a ) Circuit design (top) and truth table (bottom) for an OR gate. ( b ) Output voltage levels for all four input states of the OR gate. ( c ) Circuit design (top) and truth table (bottom) for an AND gate. ( d ) Output voltage levels for all four input states of the AND gate. Full size image An AND gate circuit can be designed on the basis of the OR gate circuit, simply by exchanging the places of the n-FET and p-FET ( Fig. 3c ). The measured output voltages for all four input combinations are shown in Fig. 3d , illustrating an excellent AND logic function. It should be noted that there are two weak '0' state outputs: an output voltage of approximately 0.02 V for input combination ( A , B )=(0, 1), and another one approximately 0.1 V for ( A , B )=(1, 0). It should also be noted that in Fig. 3 , both the OR and AND gates are composed of pairs of one p-type and one n-type pass transistor connected to each other at one source/drain node and their common gate. Depending on the desired logic function, different types of connections can be applied to the nodes of the pass transistors. Regardless of its complexity, an IC can always be constructed on the basis of the pairs of connected p-type and n-type pass transistors. Therefore, we call our PTL circuits CMOS-based CNT–PTL circuits. The main benefit of using the CMOS-based PTL circuits is that the number of transistors can be greatly reduced when compared with those based on conventional CMOS. For example, only two transistors are needed for both the OR and AND gates, whereas a total of six transistors are needed in the corresponding conventional CMOS circuit [27] , [28] . This savings in the use of transistors in ICs not only leads to higher efficiency per transistor and lower power dissipation, but also to higher speed due to the shorter signal path. Simultaneously, the performance of CMOS-based PTL circuits is not obviously degraded as a result of the small threshold voltage drop in CNT devices, because the threshold voltage of the CNT device has been suitably adjusted. In principle, by combining a CMOS NOT gate (with the basic characteristics shown in Supplementary Fig. S2 ) with basic PTL gates (for example, OR and AND), we can build hybrid CMOS/PTL circuits of any desired complexity. We first examine a full-adder circuit, which is an important combinational circuit in the ALU of a modern digital computer. A full adder adds three inputs, A , B , and a carry C i from a previous addition, and outputs a sum, SUM, and carry, C o . One way to construct a full adder is to use an exclusive-OR, or XOR, gate, which can be realised with only a pair of CMOS CNT FETs ( Fig. 4a ). A detailed analysis of all four input combinations results in a truth table ( Fig. 4a ) that is identical to that of an XOR gate. 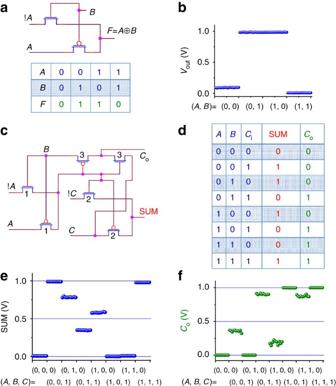Figure 4: CMOS-based pass-transistor XOR gate and a full adder. (a) Circuit design (upper) and truth table (lower) for an XOR gate. (b) Output voltage levels for all four input states of the XOR gate. (c) Circuit design and (d) truth table for a full adder, where SUM denotes summation andCodenotes carry-out. (e) Output voltage levels for SUM and the full adder for all eight input states, and (f) output voltage levels forCoand all eight input states. The measured output voltages for all four input combinations are presented in Figure 4b , in which the outputs of three combinations of ( A , B )=(0, 1), (1, 0) and (1, 1) show an almost ideal high and low logic levels. A 1-bit full adder is constructed by integrating three pairs of CMOS-based pass transistors, and its equivalent circuit diagram is shown in Fig. 4c . The truth table of the circuit is shown in Figure 4d , which is identical to that of a full adder. The measured output voltages for all eight input combinations ( A , B , C ) are shown in Fig. 4e and f , in which the outputs SUM and C 0 for all eight input combinations have similar output voltage ranges: 0–0.37 V for a logic '0' and 0.57–1 V for a logic '1', and thus match the truth table of Figure 4d . Therefore, a full adder is successfully realised experimentally on a single CNT. It is worth noting that only 6 transistors suffice to construct a 1-bit full adder with PTL, whereas a total of 28 transistors are required in a conventional CMOS circuit design. This difference represents savings of more than 78% in a transistor count, which significantly reduces the complexity of constructing a full-adder circuit. However, it should be noted that output voltages of some input combinations such as ( A , B , C )=(0, 1, 0), (0, 1, 1) and (1, 0, 0) for SUM, and ( A , B , C )=(0, 0, 1), (0, 1, 1), (1, 0, 0) and (1, 1, 0) for C o , are not as good as those for other outputs. The cause of this difference is the fact that the gain is less than 1 in all CMOS-based PTL gates, so signal degradation is unavoidable, owing to the intrinsic threshold voltage drop and fluctuations in the threshold voltages of the CNT FETs used in the circuit ( Supplementary Fig. S1b shows that the threshold voltages range from −0.33 V to 0.01 for the p-FETs and from −0.14 V to 0.46 V for the n-FETs) that arise from process nonuniformity [13] , [20] ; these voltages may be further magnified in multi-stage cascading gates. Figure 4: CMOS-based pass-transistor XOR gate and a full adder. ( a ) Circuit design (upper) and truth table (lower) for an XOR gate. ( b ) Output voltage levels for all four input states of the XOR gate. ( c ) Circuit design and ( d ) truth table for a full adder, where SUM denotes summation and C o denotes carry-out. ( e ) Output voltage levels for SUM and the full adder for all eight input states, and ( f ) output voltage levels for C o and all eight input states. Full size image The degraded output in multi-stage circuits can be restored to its ideal value by simply cascading a CMOS inverter with a gain larger than 1. As shown in Fig. 5a , when connecting a CMOS inverter to the output of a PTL XOR gate (or a semi-adder), the degraded output high level (at approximately 0.67 V) for the input combination ( A , B )=(0, 1) from the XOR gate is converted to an almost ideal low level (approximately 0.02 V, Fig. 5b ). Alternatively, the CMOS inverter can also be used to drive a PTL circuit such as the XOR gate, providing a performance similar to that using an ideal voltage source ( Fig. 5c and d ). Therefore, a CMOS inverter with a voltage gain much larger than 1 can be used in combination with PTL circuits to provide signal gain and restore the degraded signal, and to drive the next stage of the PTL gate, that is, the CNT-based PTL circuits can be used in combination with CMOS circuits to provide more reliable and complicated logic ICs without introducing any additional fabrication process. 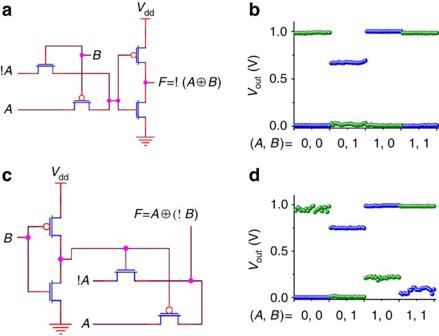Figure 5: CMOS and PTL hybrid circuits. (a) Circuit design for an XOR gate with a cascading CMOS inverter. (b) Output voltage levels for all four input states of the XOR gate without (blue spheres) and with (green spheres) a cascading CMOS inverter. (c) Circuit design for an XOR gate with a driving CMOS inverter. (d) Output voltage levels for all four input states of the XOR gate without (blue spheres) and with (green spheres) a CMOS inverter as its driving circuit. Figure 5: CMOS and PTL hybrid circuits. ( a ) Circuit design for an XOR gate with a cascading CMOS inverter. ( b ) Output voltage levels for all four input states of the XOR gate without (blue spheres) and with (green spheres) a cascading CMOS inverter. ( c ) Circuit design for an XOR gate with a driving CMOS inverter. ( d ) Output voltage levels for all four input states of the XOR gate without (blue spheres) and with (green spheres) a CMOS inverter as its driving circuit. Full size image MUX and DEMUX circuits are key components in memory and data manipulation circuits for digital ICs [27] . A two-to-one MUX circuit is designed with the CMOS-based PTL configuration, as shown in Fig. 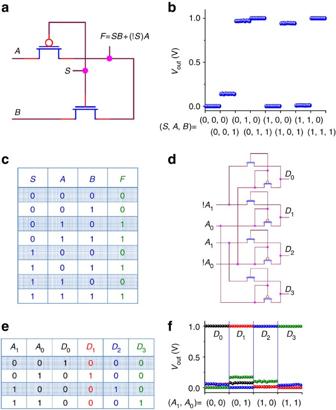Figure 6: CMOS-based two-to-one MUX and two-to-four DEMUX. (a) Circuit design for a PTL two-to-one MUX, whereSis the input control signal. (b) Experimentally measured output voltage levels for all eight input combinations of (S,A,B), and (c) the truth table of the two-to-one MUX. (d) Circuit design and (e) truth table of a PTL two-to-four DEMUX. The four outputs (D0toD3) are selected by the combinations of (A0,A1). (f) Experimentally measured output voltage levels of the two-to-four DEMUX for all four input states of (A1,A0). 6a , and the measured output voltages of the MUX circuit for all input combinations ( S , A , B ) are shown in Figure 6b . The truth table of the circuit, summarised in Figure 6c , is identical to that of a MUX. That is, A is selected as an output when S =0, whereas B is selected when S =1. The DEMUX circuit is the opposite of the MUX circuit, allowing the switching of an input to one of the many possible output lines. Figure 6d illustrates the design of a two-to-four DEMUX circuit, which consists of four AND gates connected in parallel. The DEMUX circuit works correctly, as shown in Figure 6f , in accordance with the truth table of Fig. 6e . In particular, the selected outputs from D 0 to D 3 show ideal logic '1' values without obvious degradation, and are thus competent to select and drive the next-stage circuit. Figure 6: CMOS-based two-to-one MUX and two-to-four DEMUX. ( a ) Circuit design for a PTL two-to-one MUX, where S is the input control signal. ( b ) Experimentally measured output voltage levels for all eight input combinations of ( S , A , B ), and ( c ) the truth table of the two-to-one MUX. ( d ) Circuit design and ( e ) truth table of a PTL two-to-four DEMUX. The four outputs ( D 0 to D 3 ) are selected by the combinations of ( A 0 , A 1 ). ( f ) Experimentally measured output voltage levels of the two-to-four DEMUX for all four input states of ( A 1 , A 0 ). Full size image A latch is a circuit that has two stable states and can be made to change state by applying signals to one or more control inputs. Although it is not necessary for an ALU, a latch circuit is an important storage element in sequential logic units and thus in a central processing unit. 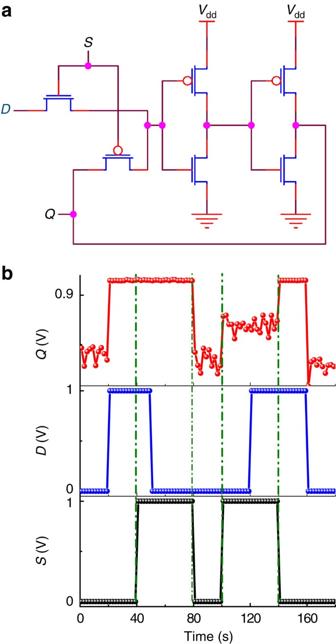Figure 7: Design and characteristics of a CNT-based D-latch circuit. (a) Circuit design with a hybrid CMOS–PTL configuration and (b) output,Q, waveforms (red), and corresponding clock (S, black) and data (D, blue) inputs. Figure 7a presents the design of a D -latch circuit with a PTL configuration, and Fig. 7b presents the relevant output ( Q ) waveforms (red) and corresponding sets of clock ( S , black) and data ( D , blue) inputs. The output Q is seen to follow the input data D when the clock S is in logic state zero during the time intervals (0, 40 s), (80, 100 s) and (140, 180 s). However, the output Q retains its previous value when S is switched into logic state one during the intervals (40, 80 s) and (100, 140 s). It should be noted that the time response of this latch circuit is slow, on the order of tens of microseconds; this is due largely to the large RC delay induced by the large capacitance coupling between the measurement pads and the conducting substrate, and the intrinsically small current of a single CNT channel. Figure 7: Design and characteristics of a CNT-based D-latch circuit. ( a ) Circuit design with a hybrid CMOS–PTL configuration and ( b ) output, Q , waveforms (red), and corresponding clock ( S , black) and data ( D , blue) inputs. Full size image It is well known that a good circuit configuration at the architectural level should take full advantage of the component device properties at the physical level. Here, we summarise the advantages of CNT-based PTL circuits. First, the number of transistors can be greatly reduced if a circuit with a desired function is designed with a PTL configuration when compared with that using the usual CMOS configuration. Reducing the number of transistors in an IC not only leads to higher efficiency per transistor, but also to higher speed and/or lower static power dissipation overall. Second, the major drawback of conventional Si-based PTL circuits—threshold voltage drop—is largely avoided in our CMOS-based CNT PTL circuits, because of the readily adjustable threshold voltage of the CNT FET. Moreover, benefitting from the near-zero threshold voltages of both the p- and n-type FETs, the power supply for these PTL circuits can be scaled down to as low as 0.4 V, even with devices having gate lengths as large as approximately 1.0 μm. The results in Fig. 8 demonstrate that the CNT-based PTL circuits such as OR ( Fig. 8a and b ) and AND ( Fig. 8c and d ) gates work properly at V DD =0.4 V ( Fig. 8b and d ). Third, although the signal gain is less than 1 in typical PTL circuits, CNT CMOS inverters with gains much greater than 1 can be cascaded at the outputs of CNT PTL circuits to provide signal amplification. In principle, CNT-based PTL/CMOS hybrid circuit configurations can be used to construct all types of complicated digital ICs, including sequential circuits such as the latch circuit shown in Fig. 7 . Last, but importantly, PTL circuits present better immunity against fluctuations in the threshold voltages of the constituent devices than CMOS circuits (as detailed in the Methods section). In CMOS circuits, the power supply at V DD is applied to pair(s) of n- and p-type FETs, and it is required that V DD should be larger than the sum of the absolute values of V th for both the p-FET and n-FET, that is, V DD >| V thp |+| V thn |. In PTL circuits, V DD is applied only on one FET (an n-type or a p-type), and V DD is thus only required to be larger than either V thn (for the n-FET) or V thp (for the p-FET). Therefore, the required power supply voltage in PTL circuits can be made much smaller than that in conventional CMOS circuits. For CNT-based PTL circuits, only a single power supply operating at V DD =1.0 or 0.4 V is required to power the entire circuit. Compared with other nano-ICs based on CNTs or nanowires requiring higher voltages or multiple power supplies [17] , [18] , [19] , [21] , [22] , [23] , [24] , [25] , [26] , our CMOS-based CNT PTL circuits offer a significant simplification of circuit design and reduced power dissipation. 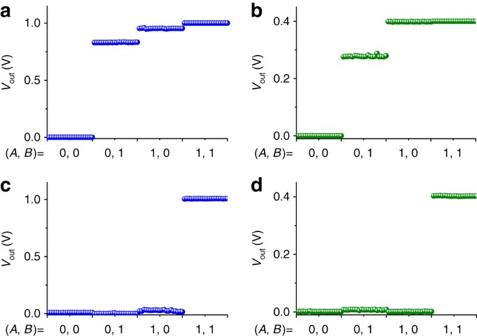Figure 8: Performance of CMOS-based PTL gates for different supply voltages. Output voltage levels for all four input states of an OR gate at (a)VDD=1.0 and (b) 0.4 V. Output voltage levels for all four input states of an AND gate at (c)VDD=1.0 and (d) 0.4 V. Figure 8: Performance of CMOS-based PTL gates for different supply voltages. Output voltage levels for all four input states of an OR gate at ( a ) V DD =1.0 and ( b ) 0.4 V. Output voltage levels for all four input states of an AND gate at ( c ) V DD =1.0 and ( d ) 0.4 V. Full size image Although the intrinsic speed of CNT-based circuits is expected to be very fast and may potentially surpass that of silicon CMOS circuits, because the CNT channel material has extremely high mobility [11] , [13] , experimentally, this high speed has not been realised owing to several parasitic effects [17] , [18] , [19] , [20] , [21] . These effects originate mainly from parasitic capacitances, which are further magnified by the well-known disadvantage of CNT FETs, that is, a small driving current when compared with that of conventional silicon devices. The major parasitic capacitances in CNT FETs include that between the gate electrode and the source/drain electrodes and that between the metallic parts (for example, contacts, interconnects and test pads) and the silicon substrate. These parasitic capacitances may in principle be significantly reduced by optimising the device structure [15] and shrinking the contact width of the source and/or drain, or by adopting an array of aligned CNTs as the channel [32] . Moreover, the parasitic capacitance between the metallic parts and the silicon substrate can be completely eliminated when an insulating substrate such as quartz, glass or plastic is used to replace the silicon [22] , [23] , [24] . The CNT-based, high-performance CMOS FETs are fabricated with a doping-free approach, in which threshold voltages for both the n- and p-type devices are adjusted to overlap near zero by selecting a suitable metal for the top gate. High-performance ICs are designed and realised with the PTL configuration, significantly reducing the number of transistors in these ICs compared with that of the conventional CMOS circuits. Combining the advantages of both the PTL configuration and the superb properties of the CNT CMOS devices, the major drawback of conventional Si-based PTL circuits—threshold voltage drop—is largely avoided, and the basic logic gates, including OR, AND and XOR, are realised with ideal high and low logic states. By incorporating a CMOS inverter with a gain much greater than one in the PTL circuits, PTL/CMOS hybrid circuits are constructed with signal gains that are not possible with pure PTL circuits, making it feasible to construct any type of complicated logic IC reliably. In addition, more complex functional units such as a full adder, and MUX and DEMUX circuits are successfully demonstrated on individual CNTs. The realisation of these circuits is sufficient for the construction of a nano-ALU. Fabrication of the devices and circuits Ultra-long SWCNTs were directionally grown on n-doped silicon wafers covered with a 500 nm, thermally grown SiO 2 layer via catalytic chemical vapour deposition [33] . Semiconducting SWCNTs were identified and selected via field-effect measurements, using the substrate as the back gate. Source ( S ) and drain ( D ) electrodes for the p-FETs were first patterned and formed via electron beam lithography, followed by evaporating an 80-nm Pd film and a standard lift-off process. The gate window was then patterned via the electron beam lithography, and a 12-nm HfO 2 film with a dielectric constant of approximately 18 was grown by atomic layer deposition at 90 °C, followed by the deposition of a 10-nm Pd film by e-beam evaporation. A standard lift-off process was used to form a self-aligned HfO 2 /Pd gate stack to complete the fabrication of the p-type CNT FETs. The fabrication of the n-FETs was similar to that of the p-FETs, but Sc was used instead of Pd for the S/D contacts. All of the FETs in this study were designed with a channel length of ∼ 1 μm. Finally, another bilayer of Ti/Au was patterned and used as interconnecting wires between the n-type and p-type FETs for external measurements. All devices and circuits were measured using a Keithley 4200 semiconductor analyser and signal sources through a probe station in air. Threshold voltage engineering As is widely known, the threshold voltage of a CNT FET is very difficult to control precisely [21] . The threshold voltage of an as-fabricated top-gate p-type CNT FET with a Ti-gate electrode is typically negative and is approximately −0.5 V (represented by the blue curves in Supplementary Fig. S1a) , whereas that of an n-type CNT FET is slightly negative [13] . To realise a symmetric CMOS inverter with a low-voltage power supply, for example, V DD =1 V, threshold voltages for both the p-type and n-type CNT FETs must be shifted in the positive direction to centre them at approximately 0 V. We previously demonstrated [13] that the threshold voltage of a CNT FET is proportional to the work function of the top gate metal, suggesting that the threshold voltage may be moved toward the more positive values by using metals with higher work functions. In this study, we used Pd as the top gate metal, which results in a reasonable threshold voltage distribution of approximately 0 V, as shown in Supplementary Fig. S1b . It should be noted that only one type of gate metal is used here. In principle, however, different metals may be used for the n- and p-FETs, which would result in overlapping threshold distributions near zero. CMOS-based PTL circuit design OR gate . The design of the OR gate is shown as an equivalent circuit in Figure 3a . Input A is applied to a p-type pass transistor, and input B is applied not only to the n-type pass transistor, but also to the common gate of the pair of pass transistors. When input B is a logic '1', which turns the n-type pass transistor on and the p-type transistor off, the output F is the same as B , which is a logic '1', regardless of the value of input A . When input B is a logic '0', which turns the n-type pass transistor off and the p-type transistor on, the output F is the same as input A . AND gate . The design of the AND gate is shown as an equivalent circuit in Figure 3c . Input A is applied to an n-type pass transistor, and input B is applied not only to the p-type pass transistor, but also to the common gate of these two pass transistors. When input B is a logic '1', which turns the n-type pass transistor on and the p-type transistor off, output F is the same as input A . When input B is a logic '0', which turns the n-type pass transistor off and the p-type transistor on, the output F is the same as input B , which is a logic '0', regardless of the value of input A . XOR gate . The XOR gate is very similar to the AND gate, but without a connection of the common gate of the two FETs to the source of the p-type pass transistor ( Fig. 4a ). When input B is a logic '1', which turns the n-type pass transistor on and the p-type transistor off, the output F is the same as input ! A (the inverse of A ). When input B is a logic '0', which turns the n-type pass transistor off and the p-type transistor on, the output F is the same as input A . Full adder . The design of a full adder is shown as an equivalent circuit in Figure 4c . The output of the first stage ( i =1) XOR logic, A B , is connected to the gate of the CMOS-based pair of pass transistors labelled (3, 3) to decide whether to pass input B ( A also works here) or input C for a carry-out output, C o . When the XOR logic of A and B outputs a logic '0', there are two different possible cases: ( A , B )=(0, 0) and ( A , B )=(1, 1). The former may not produce a carry-out, whereas the latter must produce a carry-out. In other words, C o depends only on input A or B when the output of ( A B ) is 0, regardless of the value of input C . In the cases of ( A , B )=(0, 1) and ( A , B )=(1, 0), C o depends only on input C , because if C is a logic '1' ('0'), the carry-out is a logic '1' ('0'). In the circuit design of the full adder, there are two outputs, that is, SUM and C o , representing the sum-mation and the carry-out of the inputs A + B + C , respectively, with the logic relations SUM= A B C and C o = B (! ( A B )) + C ( A B ). Although C o = B (! ( A B ))+ C ( A B ) is complex and different from the common expression of C o = AB + BC + CA in form, their functions are equivalent. Multiplexer . The MUX circuit is designed in the CMOS-based PTL configuration with only one pair of CMOS CNT FETs, as shown in Figure 6a . The control input S , which is applied to the common gate of the pass transistors, denotes the control input signal that decides which input is selected. When S is a logic '1', which turns the n-type pass transistor on and the p-type transistor off, the output F is the same as input B , regardless of the value of input A , that is, input B is selected to pass through. When input S is a logic '0', which turns the n-type pass transistor off and the p-type transistor on, input A is then selected to pass through to the output F . How to cite this article: Ding, L. et al . CMOS-based carbon nanotube pass-transistor logic integrated circuits. Nat. Commun. 3:677 doi: 10.1038/ncomms1682 (2012).